Small-molecule inhibitors targeting INK4 protein p18INK4Cenhanceex vivoexpansion of haematopoietic stem cells Among cyclin-dependent kinase inhibitors that control the G1 phase in cell cycle, only p18 and p27 can negatively regulate haematopoietic stem cell (HSC) self-renewal. In this manuscript, we demonstrate that p18 protein is a more potent inhibitor of HSC self-renewal than p27 in mouse models and its deficiency promoted HSC expansion in long-term culture. Single-cell analysis indicated that deleting p18 gene favoured self-renewing division of HSC in vitro . Based on the structure of p18 protein and in-silico screening, we further identified novel small-molecule inhibitors that can specifically block the activity of p18 protein. Our selected lead compounds were able to expand functional HSCs in a short-term culture. Thus, these putative small-molecule inhibitors for p18 protein are valuable for further dissecting the signalling pathways of stem cell self-renewal and may help develop more effective chemical agents for therapeutic expansion of HSC. Stem cells are capable of self-renewal and multi-lineage differentiation, thereby offering a major cellular source for regenerative and transplant medicine. However, the full therapeutic potential of human haematopoietic stem cell (HSC) has not yet been achieved. It is necessary to determine which combination of growth factors is optimal for net HSC expansion in vitro and what methods can effectively enhance the intrinsic self-renewing properties of HSC in vivo . The ultimate success of HSC expansion in vitro and efficient repopulation of the haematopoietic/immune system in vivo will require potent, yet specific, biological or chemical agents. These agents can provide greater insights into the downstream signalling pathways of HSC self-renewal in response to microenvironmental cues. The G1 phase of the mammalian cell cycle is a critical interface in which the somatic stem cell fate may be determined. Accumulating evidence indicates that important G1 regulators, the cyclin-dependent kinase (CDK) inhibitors (CKIs), including p16 INK4A , p18 INK4C , p21 Cip1/Waf1 , p27 kip1 and p57 kip2 , are involved in stem cell regulation [1] , [2] , [3] , [4] . However, lifting these cell-cycle ‘brakes’ appears to have different outcomes in stem cells. Later studies also showed that p57, in cooperation with p27, governed HSC quiescence by regulating the cellular localization of the Hsc70/cyclin D1 complex under homoeostasis [3] , [4] . p18, a member of the INK4 CKI family, regulates the G1 phase by inhibiting CDK4/6 (ref. 5 ). We previously demonstrated a significant increase of adult HSC self-renewal in the absence of p18 gene in vivo [6] . Subsequently, we showed that p18 absence overcame the exhaustion of HSCs in serial transplantation over the course of 3 years [7] . Notably, the role of p18 in HSCs appears to be distinct, as p21 and p18 have opposite effects [7] and p16 has an age-dependent effect on the durability of HSCs in vivo [8] . A study by Broxmeyer et al . [9] reported a decrease in the number of haematopoietic progenitor cells (HPCs) in p18 −/− mice, as measured by the colony-forming units. A unique, yet relatively specific role of p18 in HSCs was also indicated by studies from other groups. In contrast, Bowie et al . [10] reported that p18, but not other CKIs, mediates the higher responsiveness of fetal HSCs to stem cell factor (SCF), thereby explaining their higher potential for self-renewal than HSCs from adult bone marrow (BM). Sirin et al . demonstrated that p18, but not p19, p21 or p27, mediates the effect of Nurr1, a nuclear receptor transcription factor, in maintaining HSC quiescence [11] . Among all CKIs tested in HSCs, p27 was also claimed to inhibit HSC self-renewal because competitive repopulating units were increased in p27 −/− mouse BM [12] . This finding contradicted an earlier report showing p27 to have a more specific inhibitory effect on HPCs [13] . Based on distinct measurements in different studies, p18 seems to be stronger than p27 as an inhibitor of HSC self-renewal in young mice [6] , [13] . However, a direct comparison between p18 and p27 on the effects on HSCs has not been performed. Moreover, effects of p18 on haematopoietic cell proliferation, especially its direct effect on self-renewing division of HSC at single-cell level, remain to be further defined. These analyses would provide a basis for the development of specific small-molecule agents for potential HSC expansion. We now report that the effect of p18 absence is superior to p27 absence with respect to HSC self-renewal in vivo . The enhanced engraftment of transplanted HSCs in the absence of p18 is attributable to increased self-renewing division instead of a general increase of haematopoietic cell proliferation. Based on these new data and previous findings, we developed putative small-molecule inhibitors that target p18 for HSC manipulations. The compounds were first identified using in-silico three-dimensional (3D) database docking screening, and then biologically validated in vitro and further confirmed by p18 knockout (p18 −/− ) mouse model in vivo . Long-term culture and transplant assays for HSCs demonstrated the effectiveness of two lead compounds on HSC growth. The specificity of these compounds was further confirmed with p18 −/− haematopoietic cells ex vivo . Our discovery of small-molecule inhibitors that are likely specific for p18 provides valuable chemical probes to further dissect the signalling pathways of HSC self-renewal. Our findings may ultimately lead to the development of more specific chemical agents for therapeutic HSC expansion. A dominant effect of p18 over p27 on the inhibition of HSC self-renewal Given the fact that p18 seems to be a stronger inhibitor of HSC self-renewal than p27 in young mice [6] , [13] , and in order to directly compare the impact of p18 with p27 on the long-term repopulating ability of HSCs, we performed a competitive bone marrow transplantation (cBMT; Fig. 1a ). One year after transplantation, p27 −/− BM nucleated cells (BMNCs) outcompeted p27 +/+ BMNCs by 1.8-fold, whereas p18 −/− BMNCs outcompeted p18 +/+ BMNCs by a 10-fold margin ( Fig. 1b ). We thus estimated that there were five times more functional HSCs after p18 −/− transplantation than after p27 −/− transplantation. The self-renewal potential of HSCs was examined by performing a secondary transplantation in which primary transplanted p18 −/− or p27 −/− BMNCs were equally mixed with wild-type BMNCs, as previously described [7] ( Fig. 1c ). Notably, although p18 −/− BMNCs continued to outcompete p18 +/+ BMNCs in the secondary recipients, confirming our previous observation [6] , p27 −/− BMNCs did not. In the primitive cell compartment (CD34 − Lin − c-Kit + Scal + population, CD34 − LKS), the p18 −/− genotype dominated the wild-type genotype by 23-folds. In contrast, this ratio was 0.1 and 0.5 in the p27 +/+ and p27 −/− re-transplanted groups, respectively ( Fig. 1d ). Based on the immuno-phenotypic data obtained by flow cytometry and the cellularity of the BM, we estimated that transplanted p18 −/− HSCs (as defined by the CD34 − LKS immunophenotype) had undergone a 230-fold expansion. 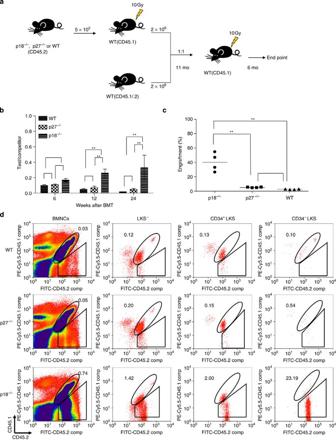Figure 1: cBMT using knockout versus wild-type cells. (a) Experimental design of the bone marrow transplantation study. 5 × 106p18−/−, p27−/−or wild-type BMNCs (CD45.2+) were injected into recipients of CD45.1 backgrounds. Eleven months (mo) after BMT, all recipients were fully reconstituted by donor-derived haematopoiesis. We then challenged transplanted HSCs (pooled from primary recipients) with an equal number (2 × 106) of un-manipulated wild-type BMNCs and transplanted them into secondary recipients (n=10). Reconstitution levels in secondary recipients were assayed for 6 months, after which the recipients were killed and subjected to flow cytometry to analyse multi-lineage haematopoietic development. (b) The ratio of test versus competitor cells. The Student’st-test was used to compare the difference among the three groups (n=10) at different time points. (c) Overall engraftment levels in BM of secondary recipients. Only p18−/−re-transplanted HSCs reconstituted the host robustly (P<0.01,n=4). (d) Relative representation in haematopoietic stem/progenitor subsets. These panels show the contribution of both transplanted HSCs and un-manipulated HSCs at different stages of haematopoiesis. Here, the CD45.2 population was contributed by transplanted cells, whereas double positive populations were contributed by un-manipulated cells. The values in the corner show the ratio of CD45.2 versus double positive cells. In the wild-type group, fresh HSCs dominated at both the progenitor and stem cell level. The CD34–LSK cells are largely responsible for long-term engraftment in transplanted animals. Data sets were analysed using one-way analysis of variance (GraphPad Prism v6.0). All data represent mean±s.d. *P<0.05, **P<0.01. In contrast, there was only a 6.9- and 2.5-fold expansion of p27 −/− and p27 +/+ HSCs in the secondary recipients, respectively ( Table 1 ). Considering that for every 2 × 10 6 co-transplanted BMNCs, the input number of long-term hemopoietic stem cells (LT-HSCs) from p18 −/− mice was 1.5–2 times more than that from p27 −/− mice (data not shown), we estimated that there were 16 times more HSCs generated in p18 −/− repopulated mice than in p27 −/− repopulated mice 1 year after transplantation. These results were highly consistent with the results from direct comparison between p18 −/− and p27 −/− BMNCs (from CD45.1 and CD45.2 congenic strains) that were co-transplanted into the same recipients ( Supplementary Fig. 1a–c and Supplementary Table 1 ). Figure 1: cBMT using knockout versus wild-type cells. ( a ) Experimental design of the bone marrow transplantation study. 5 × 10 6 p18 −/− , p27 −/− or wild-type BMNCs (CD45.2 + ) were injected into recipients of CD45.1 backgrounds. Eleven months (mo) after BMT, all recipients were fully reconstituted by donor-derived haematopoiesis. We then challenged transplanted HSCs (pooled from primary recipients) with an equal number (2 × 10 6 ) of un-manipulated wild-type BMNCs and transplanted them into secondary recipients ( n =10). Reconstitution levels in secondary recipients were assayed for 6 months, after which the recipients were killed and subjected to flow cytometry to analyse multi-lineage haematopoietic development. ( b ) The ratio of test versus competitor cells. The Student’s t -test was used to compare the difference among the three groups ( n =10) at different time points. ( c ) Overall engraftment levels in BM of secondary recipients. Only p18 −/− re-transplanted HSCs reconstituted the host robustly ( P <0.01, n =4). ( d ) Relative representation in haematopoietic stem/progenitor subsets. These panels show the contribution of both transplanted HSCs and un-manipulated HSCs at different stages of haematopoiesis. Here, the CD45.2 population was contributed by transplanted cells, whereas double positive populations were contributed by un-manipulated cells. The values in the corner show the ratio of CD45.2 versus double positive cells. In the wild-type group, fresh HSCs dominated at both the progenitor and stem cell level. The CD34 – LSK cells are largely responsible for long-term engraftment in transplanted animals. Data sets were analysed using one-way analysis of variance (GraphPad Prism v6.0). All data represent mean±s.d. * P <0.05, ** P <0.01. Full size image Table 1 Estimated function per HSC from primary and secondary recipients. Full size table Enhanced self-renewing division of p18 −/− HSC As p18 is an inhibitor of CDK4/6, a regulator of the G1 cell-cycle phase, a general increase of haematopoietic cell proliferation may improve long-term engraftment [6] . To test this effect, we measured the cell cycling fraction in different haematopoietic subpopulations by 5-bromodeoxyuridine (BrdU) incorporation in vitro and in vivo . There was no significant difference in BrdU uptake between the p18 −/− and p18 +/+ groups ( Supplementary Fig. 2a,b ). Data from these BrdU assays in both transplanted and non-transplanted mice strongly indicate that a general increase of haematopoietic cell proliferation is not responsible for the improved engraftment in the absence of p18. To vigorously assess the proliferative rate of the stem cells with a more primitive HSC phenotype, we also examined CD34 − LKS cells using a single-cell culture system. There was no significant difference in the rate of cell division between the p18 −/− and p18 +/+ groups ( Supplementary Fig. 2c–f ). To determine the homing ability of transplanted HSCs, we measured the total number of homed cells (CD45.2) in the BM 17 h after Lin − c-Kit + Scal + cells were injected into the recipients. The absolute number of homed cells in the BM did not significantly differed between p18 −/− and p18 +/+ groups ( Supplementary Fig. 2g ). The cell-cycle status of HSCs (CD150 + CD48 − LKS) was further examined. There was no statistical difference in the fraction of viable cells in each phase of the cell cycle between p18 +/+ and p18 −/− groups ( P >0.05, n =5; Supplementary Fig. 2h ). Therefore, p18 deficiency does not increase the proliferative or survival rate of primitive HSCs under culture conditions, thereby suggesting a paradigm in which absence of p18 favours self-renewing division, not differentiating division. The increased self-renewing division of HSC in the absence of p18 was first explored by using an in vitro culture system. Individual daughter HSCs, after first division, were micro-manipulated and cultured to be traced for their differentiation potential in myeloid lineages, including netrophils (n), monocytes (m), erythrocytes (E) and megakaryocytes (M). According to Takano et al . [14] , the outcome of generating nmEM mixed cell populations from a single cell under this culture condition highly correlates with the long-term multi-lineage repopulating ability in vivo [14] , [15] , thereby reflecting the ‘stemness’ of an original input cell with an HSC immunophenotype (CD34 − LKS). Four experiments were performed in our study ( Fig. 2a ) [16] . In the p18 +/+ group, we analysed 74 cell pairs. Among 24 pairs that generated nmEM, three symmetric divisions (both daughter cells generating nmEM progeny) were found. In the p18 −/− group, we analysed 69 pairs, 35 of which generated nmEM and 10 symmetric divisions were observed. A statistically significant difference between the p18 +/+ and p18 −/− groups is shown, based on a paired Student’s t -test for multiple experiments ( n =4), as indicated in the graphs showing the percentage of parental HSCs ( Fig. 2b left) or paired daughter HSCs that were able to form the nmEM progeny ( Fig. 2b right). Our results thus demonstrate a significantly increased probability that p18 −/− cells generate more colonies of nmEM cells from paired daughter HSCs. 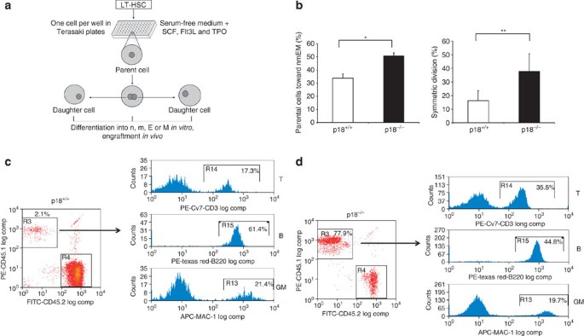Figure 2: Increased probability of symmetric self-renewing division of HSC. (a) Experimental approach of paired daughter stem cell analysisin vitroand multi-lineage engraftment of two daughter cells from a single HSC. (b) Percentage of parental HSCs committed to the nmEM lineage (left) and paired daughter HSCs able to form the nmEM progeny (right). (c) Representative recipient of the p18+/+daughter cell. (d) Representative recipient of the p18−/−daughter cell. Multi-lineage differentiation was examined by flow cytometry. GM, T and B indicate lineages for myloid, T cells and B cells, respectively. Data sets were analysed using one-way analysis of variance (GraphPad Prism v6.0). All data represent mean±s.d. in different groups. *P<0.05, **P<0.01. Figure 2: Increased probability of symmetric self-renewing division of HSC. ( a ) Experimental approach of paired daughter stem cell analysis in vitro and multi-lineage engraftment of two daughter cells from a single HSC. ( b ) Percentage of parental HSCs committed to the nmEM lineage (left) and paired daughter HSCs able to form the nmEM progeny (right). ( c ) Representative recipient of the p18 +/+ daughter cell. ( d ) Representative recipient of the p18 −/− daughter cell. Multi-lineage differentiation was examined by flow cytometry. GM, T and B indicate lineages for myloid, T cells and B cells, respectively. Data sets were analysed using one-way analysis of variance (GraphPad Prism v6.0). All data represent mean±s.d. in different groups. * P <0.05, ** P <0.01. Full size image The increased self-renewing division of HSC in the absence of p18 was further evaluated by transplantation of daughter cells from the first division of single HSCs. Individual daughter HSCs engrafted five mice in the p18 −/− group, whereas only two mice in the p18 +/+ group ( n =64 pairs each). Moreover, the mean value for engrafted mice was much higher in p18 −/− group than in p18 +/+ group (26.67%±0.35 versus 2.37%±0.004; Table 2 ). When a secondary bone marrow transplantation (BMT) was conducted, no engraftment was observed in the p18 +/+ group. In contrast, there was a considerable level of engraftment in the p18 −/− group (0.61–9.44%, n =4; Table 2 ). Admittedly, we were not able to document the multi-lineage engraftment of paired daughter HSC cells in either p18 +/+ or p18 −/− group. Nevertheless, these different assays provide definitive evidence for a direct inhibitory role of p18 in self-renewing division of HSC and enhanced haematopoietic engraftment in the absence of p18 was not due to increased general proliferation of haematopoietic cells. Table 2 Engraftment levels in recipients of daughter cells. Full size table In-sililco screening and specificity of identified p18 inhibitors Based on the strong inhibitory effect of p18 in self-renewal of HSC as shown above, we then attempted to develop small-molecule inhibitors of p18 protein for HSC expansion ex vivo . To overcome the low throughput capability of current HSC assays, we first conducted 3D database docking search to screen for virtual p18 inhibitors based on p18 protein structure and predicted binding surface cavity, using the reported protocols [17] , [18] . The 3D structural model of the p18/CDK6/cyclin ternary complex ( Fig. 3a ) was constructed according to reported X-ray crystal structures [19] , [20] . The p18 protein, with five ankyrin repeats and its surface binding cavity, is depicted in Fig. 3b . A putative ligand-binding cavity on the p18 surface was defined by the Connolly solvent-accessible surface calculation [18] with a 1.4-Å radius ( Fig. 3b ). 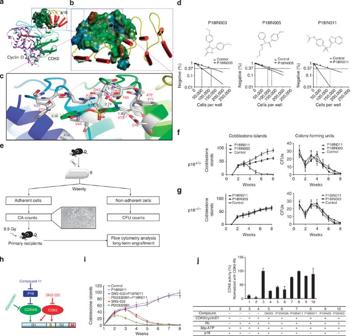Figure 3:In-silicoscreening for p18-specific small-molecule inhibitors. (a) 3D structural model of the p18/CDK6/CylinD complex (left) and the p18-binding surface cavity (right), showing that p18 (red colour) binds to CDK6 (green) at the site opposite cyclin-D (purple). (b) A docking pose of P18IN011, depicting hydrogen bonding and hydrophobic interactions between P18IN011 and the key residues of the p18 protein. (c) Putative interactions between P18IN011 and p18 residues. (d) The structure of the lead compounds and the limit dilution analysis of groups treated with different compounds. (e) Experimental design of Dexter-type long-term cultures of BMNCs. The data were from one of two experiments yielding similar results. A specific effect of p18 small-molecular inhibitors on p18+/+(f) haematopoietic cells, but not on p18−/−(g) haematopoietic cells, during long-term BM culture. Freshly isolated BMNCs from p18+/+mice or p18−/−mice were cultured in the Dexter’s culture medium presence or absence of the lead compounds and the cobblestone area (CA) number was counted each week (left). Non-adherent cells from the old medium were seeded in 0.5 ml of M3434 (StemCell Technologies) supplemented with recombinant cytokines (50 ng ml−1of SCF, 10 ng ml−1of IL-3, 10 ng ml−1of IL-6 and 3 U ml−1of EPO). The cells were plated in a 1.7-cm dish (n=5) at a fixed density. The existence of CFUs in each well was counted weekly (right). (h) A model of cell-cycle regulation by p18 and CDKs. (i) Specific dependence of p18 inhibitor compounds on CDK4/6, but not on CDK2. (j) CDK6 activity assayin vitro. Recombinant Rb fragments were used as substrates for the activated complexes of CDK6/CyclinD1. P-labelled GST-Rb was quantitatively analysed by a scintillation counter and normalized with the mean of the CDK6-Rb group. P18IN3A was used as a negative control. Data sets were analysed using one-way analysis of variance (GraphPad Prism v6.0). All data represent mean±s.d. in different groups. *P<0.05, **P<0.01. Figure 3: In-silico screening for p18-specific small-molecule inhibitors. ( a ) 3D structural model of the p18/CDK6/CylinD complex (left) and the p18-binding surface cavity (right), showing that p18 (red colour) binds to CDK6 (green) at the site opposite cyclin-D (purple). ( b ) A docking pose of P18IN011, depicting hydrogen bonding and hydrophobic interactions between P18IN011 and the key residues of the p18 protein. ( c ) Putative interactions between P18IN011 and p18 residues. ( d ) The structure of the lead compounds and the limit dilution analysis of groups treated with different compounds. ( e ) Experimental design of Dexter-type long-term cultures of BMNCs. The data were from one of two experiments yielding similar results. A specific effect of p18 small-molecular inhibitors on p18 +/+ ( f ) haematopoietic cells, but not on p18 −/− ( g ) haematopoietic cells, during long-term BM culture. Freshly isolated BMNCs from p18 +/+ mice or p18 −/− mice were cultured in the Dexter’s culture medium presence or absence of the lead compounds and the cobblestone area (CA) number was counted each week (left). Non-adherent cells from the old medium were seeded in 0.5 ml of M3434 (StemCell Technologies) supplemented with recombinant cytokines (50 ng ml −1 of SCF, 10 ng ml −1 of IL-3, 10 ng ml −1 of IL-6 and 3 U ml −1 of EPO). The cells were plated in a 1.7-cm dish ( n =5) at a fixed density. The existence of CFUs in each well was counted weekly (right). ( h ) A model of cell-cycle regulation by p18 and CDKs. ( i ) Specific dependence of p18 inhibitor compounds on CDK4/6, but not on CDK2. ( j ) CDK6 activity assay in vitro . Recombinant Rb fragments were used as substrates for the activated complexes of CDK6/CyclinD1. P-labelled GST-Rb was quantitatively analysed by a scintillation counter and normalized with the mean of the CDK6-Rb group. P18IN3A was used as a negative control. Data sets were analysed using one-way analysis of variance (GraphPad Prism v6.0). All data represent mean±s.d. in different groups. * P <0.05, ** P <0.01. Full size image A 3D virtual compound library [21] was used for the virtual screening. We identified several small molecules that have strong H-bonding and hydrophobic interactions with the p18 protein (~3 Å; Supplementary Fig. 3a ). P18IN011 (MW=332.33, Clog P 2.3) was identified as one of the virtual hits by the Surflex-dock database search ( Fig. 3c ). The docking pose shows that the chemical lead P18IN011 has extensive H-bonding interactions with key p18 residues, including its amide NH group with D76 (1.90 Å), C=O with Q43 (3.16 Å) and D67 (3.20 Å), sulfonate O=S=O with T69 (2.71 Å) and its charge interaction with R39 (charge interaction, 3.12 Å; Fig. 3c ). Hydrophobic interactions were also detected for its isoxazobenzine ring with F37 and V44 of p18, and the acetamidobenzene ring surrounded by hydrophobic residues F71, A72 and V73 of p18 in a range of 3.3–3.7 Å. The F37, R39, Q43, V44, D67 and D76 residues of p18 are known to be highly conserved, located at the p18/CDK6 interface and known to play important roles in the H-bonding or hydrophobic interactions of p18 with CDK6. The additional binding residues identified, T69, F71, A72 and V73, are exclusive for p18 based on homology modelling in comparison with other CKI proteins ( Supplementary Fig. 3b ) [20] . By blocking these key residues, a compound is predicted to disrupt the interaction of p18 with CDK6. This disruption has been confirmed by our following biological experiments. We performed the Cobblestone-Area Forming Cell (CAFC) assay with limiting dilution or bulk culture of BMNCs [6] , [7] , [13] to validate the effects of the identified p18 small-molecule inhibitors on haematopoietic cells. Cultures were treated with 20 μM of either P18IN003 or P18IN011. The CAFC frequency at day 35 (indicating the activity of HSCs) was 3.26 times more in the P18IN003-treated culture and 4.21 times more than in the P18IN011-treated culture ( Fig. 3d ), compared with control cultures. For the P18IN003A-, P18IN004- and P18IN005-treated groups (20 μM), effects on CAFC frequency were marginal ( P >0.05, n =5; Supplementary Fig. 3c ). Dose–response experiments showed that the IC50 value was 6.12 μM for P18IN003 and 3.61 μM for P18IN011. These results suggest that P18IN011 and P18IN003 could significantly increase the frequency of primitive haematopoietic cells in culture. We investigated whether the effects of p18 small-molecule inhibitors (P18IN003 and P18IN011) on haematopoietic cells are specific to the p18 protein. In the long-term culture of p18 +/+ mouse BMNCs [22] , [23] ( Fig. 3e ), there was no significant difference in CA (cobblestone area) yields in the first 4 weeks between the control group and the groups treated with p18 small-molecular inhibitors. After 5–8 weeks of culture, however, more CAs were generated after treatment with P18IN003 or P18IN011 ( P <0.01, n =5; Fig. 3f left). More CAs were generated after treatment with P18IN011 than P18IN003 at the same concentrations ( P <0.01, n =5; Fig. 3f left), whereas there was no significant difference in colony-forming unit (CFU) among the three groups ( P >0.05, n =5; Fig. 3f right). When p18 −/− mouse BMNCs were used, data were congruent with the in vitro p18 small-molecule inhibitor studies. Consistent with previous observations [6] , significantly more CAs were generated from p18 −/− BMNCs than from p18 +/+ BMNCs ( P <0.01, n =5; Fig. 3f left). For p18 −/− mouse BMNCs, however, treatment with P18IN011 or P18IN003 did not generate more CAs than the control group ( Fig. 3g left). Again, CFUs did not differ among the three groups ( Fig. 3g right). We also transplanted the cells after 8 weeks of long-term culture in the presence or absence of the compounds. There was no engraftment from the control group. In contrast, six of eight mice in the P18IN003 group and eight of eight mice in the P18IN011 group engrafted at considerable levels (12.31±2.18% and 22.06±3.01%, respectively). These data indicate that the identified p18 small-molecule inhibitors were able to sustain the function of HSCs in the culture. To further determine whether inhibition of the p18 protein by p18 putative inhibitors is specific to CDK4/6, we applied two known small-molecule inhibitors, PD0332991 (to CDK4/6) and SNS-032 (to CDK2), to p18 +/+ long-term cultures ( Fig. 3h ). The increase of CAs of BMNCs treated with P18IN011 was blocked by PD0332991, but not by SNS-032 ( Fig. 3i ). The p18 small-molecular inhibitors apparently affected haematopoietic regulation through CDK4/6 rather than through CDK2. An in vitro CDK6 activity assay in the presence of GST-p18 protein was further performed to prove the specificity of these compounds. Compound P18IN003A, a top hit from the virtual screening, which had a score of 5.62, but had no effect on CAFC frequency was used as a negative control in the CDK6 assay. Pre-incubation with P18IN011 or P18IN003 prevents GST-p18 from significantly inhibiting CDK6 activity; in the absence of p18 small-molecular inhibitors, 100 ng GST-p18 inhibited CDK6 activity by more than 70% ( Fig. 3j ). These results suggest that the binding of p18 with CDK6 can be directly blocked by the putative inhibitors. The same in vitro CDK6 activity assay was further performed with GST-p16 to test whether these p18 small-molecule inhibitors are also able to block p16 protein. The p18 inhibitors (P18IN011 or P18IN003) did not prevent GST-p16 from significantly inhibiting CDK6 activity ( Supplementary Fig. 3d ), thereby suggesting a relative specificity of these compounds for p18 protein, not other INK4 proteins such as p16. Direct effect of p18 small-molecule inhibitors on ex vivo HSC expansion Our next experiment was intended to test the direct effects of the p18 small-molecule inhibitors on purified HSCs in a short-term liquid culture. We isolated purified HSCs, cultured them in the presence of P18IN003 or P18IN011, and then determined their long-term repopulation via cBMT. Fifty CD34 − LKS cells isolated from CD45.1 mice were cultured in Iscove’s modified Dulbecco’s medium supplemented with 50 ng ml −1 SCF, 10 ng ml −1 thrombopoietin (TPO) and 1 μl dimethylsulphoxide (DMSO; blank control) or 10 μM p18 inhibitors for 3 days. The test cells, together with competitor cells (BMNCs freshly isolated from CD45.2 mice), were co-transplanted into lethally irradiated recipients ( Fig. 4a ). The engraftment of both P18IN003- and P18IN011-treated groups were significantly higher than control group ( P <0.01, n =10; Fig. 4b left) 16 weeks after transplantation. Moreover, engraftment of P18IN011-treated group was two times more than that of the P18IN003-treated group ( P <0.01, n =10). These results further confirmed that P18IN003 and P18IN011 significantly expanded the long-term repopulating ability of HSCs after the short-term culture in vitro . In addition, no predominant growth of any specific lineages was found after treated with the compounds ( Fig. 4b right). Limiting dilution analysis was performed to quantitatively compare the frequencies of functional HSCs in different groups ( Supplementary Fig. 4 ). The HSC frequency was approximately 4.2-fold higher in P18IN011 group than that in DMSO group. Similar HSC frequency was detected in the negative p18 putative inhibitor (P18IN005) and DMSO group. 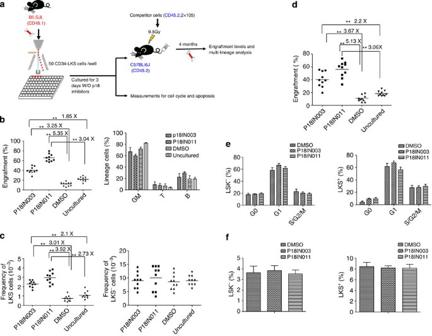Figure 4: Enhanced expansion of HSCsin vitroandex vivo. (a) Experimental design. CD34-LKS cells were sorted into 96-well plates at 50 cells per well and cultured for 3 days in the presence of SCF, TPO and the lead compound or 1 μl of DMSO. Cells from each well were mixed with 1 × 105freshly isolated BMNCs and transplanted via tail vein injection into lethally irradiated CD45.2 recipient mice. At 16 weeks after transplantation, BMNCs were stained to determine the engraftment level of donor cells. BMNCs were also stained for lineage, HSC and HPC analyses. BMNCs from recipients were further cultured in methylcellulose for CFU quantification. (b) The engraftment levels at 16 weeks after primary transplantation (left), and multi-lineage differentiation profile (right). Multi-lineage differentiation was examined by flow cytometry. GM, T and B indicate lineages for myloid, T cells and B cells, respectively. (c) Phenotypic quantification for HSC (left) and committed HPC (right) pools. (d) Secondary transplantation. (e) Flow cytometry analysis of cell cycle in LKS+cells and LKS−cells treated with inhibitor compounds or DMSO. The average percentages of G0, G1 and S/G2/M fractions in LKS−cells (left,P>0.05,n=10) and LKS+(right,P>0.05,n=10) from three experiments are summarized. (f) Detection of LKS−and LKS+cell apoptosis by 7-AAD staining. LKS+cells (right) or LKS−(left) cells treated with inhibitor compounds showed no increase in Annexin-V and 7-AAD positivity, as detected by flow cytometry (P>0.05,n=10). Data sets were analysed using one-way analysis of variance (GraphPad Prism v6.0). All data represent mean±s.d. *P<0.05, **P<0.01. W/O, with or without. Figure 4: Enhanced expansion of HSCs in vitro and ex vivo . ( a ) Experimental design. CD34-LKS cells were sorted into 96-well plates at 50 cells per well and cultured for 3 days in the presence of SCF, TPO and the lead compound or 1 μl of DMSO. Cells from each well were mixed with 1 × 10 5 freshly isolated BMNCs and transplanted via tail vein injection into lethally irradiated CD45.2 recipient mice. At 16 weeks after transplantation, BMNCs were stained to determine the engraftment level of donor cells. BMNCs were also stained for lineage, HSC and HPC analyses. BMNCs from recipients were further cultured in methylcellulose for CFU quantification. ( b ) The engraftment levels at 16 weeks after primary transplantation (left), and multi-lineage differentiation profile (right). Multi-lineage differentiation was examined by flow cytometry. GM, T and B indicate lineages for myloid, T cells and B cells, respectively. ( c ) Phenotypic quantification for HSC (left) and committed HPC (right) pools. ( d ) Secondary transplantation. ( e ) Flow cytometry analysis of cell cycle in LKS + cells and LKS − cells treated with inhibitor compounds or DMSO. The average percentages of G0, G1 and S/G2/M fractions in LKS − cells (left, P >0.05, n =10) and LKS + (right, P >0.05, n =10) from three experiments are summarized. ( f ) Detection of LKS − and LKS + cell apoptosis by 7-AAD staining. LKS + cells (right) or LKS − (left) cells treated with inhibitor compounds showed no increase in Annexin-V and 7-AAD positivity, as detected by flow cytometry ( P >0.05, n =10). Data sets were analysed using one-way analysis of variance (GraphPad Prism v6.0). All data represent mean±s.d. * P <0.05, ** P <0.01. W/O, with or without. Full size image The frequency of LKS cells and LKS − cells in CD45.1 + cells was also analysed. LKS cells in the groups treated with P18IN003 or P18IN011 were significantly higher than the control group ( P <0.01, n =10; Fig. 4c left). LKS cells were 1.3-fold more abundant in the group treated with P18IN011 than with P18IN003 ( P <0.01, n =10). In contrast, the frequency of LKS − cells did not differ significantly among the three groups ( P >0.05, n =10; Fig. 4c right). We also performed a secondary BMT to further test whether the phenotypically enlarged HSC pool in vivo is correlated with its function. The engraftment levels of the groups treated with P18IN003 or P18IN011 remained significantly higher than the level of the control group ( P <0.01, n =10). Higher engraftment occurred in the P18IN011-treated group than in the P18IN003-treated group ( P <0.01, n =10; Fig. 4d ). The cell-cycle status of HSCs and the contribution of apoptosis were examined after treatment with the p18INs for 3 days. The fraction of viable cells in each phase of the cell cycle remained unchanged after treatment with the p18 putative inhibitors ( P >0.05, n =10; Fig. 4e ). Furthermore, there is no statistical difference in the apoptotic fractions between the control, P18IN003 and P18IN011 groups ( P >0.05, n =10; Fig. 4f ). This suggests that cell proliferation and apoptosis may not be the reason for the increase of HSC self-renewal after treatment with the p18IN compounds, as similarly demonstrated in p18 −/− mice. Ex vivo expansion of human HSCs from human cord blood remains an unattained goal of clinical HSC transplantation. A variety of methods have been explored to expand HSCs ex vivo . Most techniques involve a cocktail of haematopoietic cytokines, which can often promote HSC differentiation and consequently result in depletion of HSCs. Some exceptions include the use of insulin growth factor-binding protein 2 or/and angiopoietin-like proteins in combination with SCF, TPO and fibroblast growth factor-1 (refs 24 , 25 ). In recent years, a number of small-molecule inhibitors have been developed to stimulate HSC expansion or maintenance [26] . In particular, activation of the Wnt/β-catenin pathway by glycogen synthase kinase-3 inhibitor, CHIR99021, has been explored [27] , [28] . The effect of this single agent, however, seemed to be insufficient for HSC expansion as activation of both the Wnt/β-catenin pathway and the Pten/PI3/Akt or mTOR pathways, with small molecules in conjunction with low concentrations of growth factors, was able to markedly expand HSC expansion [29] . However, this potent strategy may be complicated by tumorigenic processes that commonly involve both pathways. Noticeably, a recent study [30] reported that mouse or human HSCs can be maintained in serum-free, cytokine-free medium in the presence of CHIR99021 and the mTOR inhibitor, rapamycin, for 7 days. Although this study was the first demonstration that HSCs can be maintained in a cytokine-free culture system in vitro , net expansion of HSCs by this method was not proved. In addition, it should be noted that a previous study on SR1 (ref. 31 ) and a recent report on UM171 (ref. 32 ) were reported to be able to expand human cord blood-derived short-term HSCs and long-term HSCs, respectively. However, these compounds were shown to only affect human HSCs but not mouse HSCs. Moreover, the mechanisms underlying these reported small molecules are largely unknown. Given the fact that there are no published reports yet regarding the clinical usefulness of SR1 or UM171 so far, new studies particularly with strong biological bases as shown by our current study are still in demand. Therefore, our current study would deserve attention and further exploration with human HSCs. Problematically, acceleration of cell proliferation is often associated with functional exhaustion of HSCs [1] , [2] , [3] , [4] and thus most stimuli on cell-cycle progression have not shown to be effective in HSC expansion. p18 is potentially a good target for HSC expansion, because it does not seem to primarily affect the cell proliferation rate. Instead, it impacts the outcome of HSC division. Single HSC daughter culture and transplantation both support the increase of self-renewing division in the absence of p18, although direct evidence for the role of p18 in the balance between symmetric and asymmetric division is yet to be further obtained. It is unclear how p18 regulates symmetry of HSC division at the molecular level. In addition, the role of p18 in stem cell regulation appears to be development dependent, as our recent study suggests an opposite effect of p18 overexpression in mouse ES cells as opposed to adult stem cells or tumour cells [33] . Furthermore, p18 has not been shown to commonly associate with human cancers. Our study consistently showed that HSCs are not the direct targets for potential T-cell leukemogenesis in p18 −/− aged or transplant mice [34] . Because p18 is broadly expressed in multiple tissues, targeting p18 probably also has effects on other tissue stem cells. In summary, we have focused on the role of CKIs in stem cell regulation and found that targeting specific CKIs may yield different outcomes. p18 represents a potent and specific target for enhancing the self-renewal property of HSC. Development of more effective p18 inhibitors or its combinations with other HSC expansion agents may offer effective agents for HSC expansion in the future. Mice All the p27 or p18 heterozygous or homozygous mice used for cBMT studies had a C57BL/6 (CD45.2) background or the congenic B6.SJL-Ptprc a Pep3 b /Boy (CD45.1) background (more than ten generations backcrossed onto congenic background from the original C57BL/6; 129/Sv mixed background). The donor mice for cBMT were 3- to 6-month-old males and the recipients were 2- to 3-month-old females (the same age was used between wild-type and knockout mice for each experiment). All the procedures involving animal experiments were approved by the Institutional Animal Care and Use Committee at the University of Pittsburgh and also the Institute of Hematology of the Chinese Academy of Medical Science. Phenotypic analysis and cell sorting For the quantification of HSC versus HPC in the transplant mice, different subsets were used, defined by c-Kit and Sca-1 within the Lin-cell populations (LKS). CD34-LKS was used to quantify LT-HSCs in vivo . For the analyses of a single HSC or daughter HSC in vitro and in vivo (single-cell transplant assay), a more stringent protocol was used to isolate primitive HSC based on the RhdaminlowCD34-LKS or CD150+CD48-CD34-LKS phenotypes. The staining methods are described in our published protocols [35] , [36] . Briefly, BM cells were flushed from the tibias, femurs and iliums in PBS+2 mM EDTA buffer supplemented with 2% heat-inactivated bovine serum (Gibco). Then cells were filtered through nylon screen (100 μm) to get a single-cell suspension. Antibodies against CD34 (Clone:RAM34), FLK2/FLT32 (Clone:A2F10.1), c-Kit(Clone:2B8), Sca-1(Clone:D7), FcγRII/III (Clone:93), CD3 (Clone:145-2C11), B220 (Clone:RA3–6B2), CD11b(Mac-1) (Clone: M1/70), Gr-1 (Clone: RB6–8C5), CD4 (Clone: GK1.5), CD8 (Clone: 53–6.7), Ter119 (Clone: TER119), IL-7Rα (CD127) (Clone: A7R34), CD45.1 (Clone: A20), CD45.2 (Clone: 104)and CD48(HM48-1) were from eBioscience. Antibody against CD150 (TC15-12F12.2) was from BioLegend. The lineage cocktail contained Ter119, Gr-1, Mac-1, B220, CD3, CD4 and CD8 antibodies. Flow cytometry was performed with FACS Aria III or LSR II (BD Biosciences). Cell-cycle analysis and apoptosis assays BrdU was administered continuously to the mice, via their drinking water, at a concentration of 0.5 mg ml −1 for 13 weeks. Transplant mice received intra-peritoneal injections of 100 μg g −1 BrdU 16 h before killing. BMNCs were collected at different time points to stain for multiple cell surface markers and BrdU. The BrdU labelling kit for flow cytometry (BD Pharmingen) was used according to the manufacturer’s protocol in conjunction with the phenotypic analysis described in the ‘phenotypic analysis and cell sorting’ section. The G0 versus G1 analysis involving PY staining was detailed in our published protocol [36] . For the apoptosis assay, BMNCs treated with the P18INs compounds or DMSO for 3 days were isolated and stained with a mixture of PE-Cy7-conjugated lineage antibodies, PE–Annexin-V and congenic markers (BD Bioscience). The proportion of apoptotic cells was determined using BD-LSR flow cytometry. Single-cell assays Rhdamin low CD34 − LKS or CD150 + CD48 − CD34 − LKS cells were sorted into Tarasaki plates at one cell per well using the High-Speed MoFlo or BD influx Cell Sorter. Each well contained 10 μl of BIT9500 medium supplemented with 50 ng ml −1 Flt3 ligand (Flt3-L), 100 ng ml −1 SCF and 20 ng ml −1 TPO. The first division of a single cell was followed within 72 h after seeding. Two daughter cells generated by one single cell were separated through micromanipulation for the in vitro and in vivo studies. In vitro differentiation: paired daughter cells were transferred into the serum-free medium containing a cytokine combination of 100 ng ml −1 of SCF , 25 ng ml −1 of TPO, 10 ng ml −1 of interleukin (IL)-3 and 10 ng ml −1 of erythropoietin (EPO). The colony-forming rate and the potential of differentiation into granulocytes (n), monocyte/macrophages (m), erythroblasts (E) or megakaryocytes (M) were recorded at day 10 in culture. In vivo transplantation: paired daughter cells, along with competitive cells, were separately injected into lethally irradiated mice (one daughter cell per mouse) and engraftment levels were monitored at different times after transplantation, as described in the ‘HSC transplantation’ section. HSC transplantation In all the transplantation experiments, female recipients aged 2–3 months were irradiated with 9.0 or 10 Gy on the day before transplantation. Varied numbers of donor test cells along with competitive cells in a congenic background were injected into the tail vein. Specific doses of transplanted cells were described in the legend of the related figures. The single-cell manipulation for daughter HSCs is described in the ‘Single-cell assays’ section. Long-term BM co-culture Freshly isolated BMNCs from mice, 6–8 weeks old, were plated in a 24-well plate with 1 ml Dexter’s medium at a density of 2 × 10 6 cells per ml in the absence or presence of different doses of the tested compounds. The culture was maintained at 33 °C with 5% CO 2 . The number of CAs was counted weekly. The medium was also replaced with half fresh medium on a weekly basis. Non-adherent cells from the old medium were collected, counted and then seeded in 0.5 ml M3434 (methylcellulose medium, StemCell Technologies) supplemented with recombinant cytokines (50 ng ml −1 SCF, 10 ng ml −1 IL-3, 10 ng ml −1 IL-6 and 3 U ml −1 of EPO). The cells were plated in a 1.7-cm dish (× 5) at a density of 1.5 × 10 4 cells per ml. The existence of CFUs in each well was counted under an inverted microscope once each week for 5 consecutive weeks and reported as total colony yield or colony number in a specific lineage. At 8 weeks after the long-term culture, 2–10 × 10 5 cells with non-adherent and adherent populations from two wells were transplanted into lethally irradiated mice (CD45.1) to confirm the long-term repopulation potential of ex vivo expanded or maintained HSCs. For the limiting dilution analysis of the test cells, different limiting doses were plated on the irradiated stroma in 96-well plates containing 200 μl of M5300 medium (StemCell Technologies) supplemented with 10 −6 M hydrocortisone. Small-molecule compounds were added to the co-culture system at different doses. Half of the medium in each well was replaced with fresh medium containing the test compounds weekly. The existence of CA in each well was evaluated under an inverted microscope at weekly intervals for 5 weeks. Based on the Poisson distribution of the negative wells, the frequency of long-term initiating cells was calculated with L-Calc software (StemCell Technologies). CFU assay Cells were plated in triplicate in M3434 medium (StemCell Technologies) and different types of CFUs were counted at day 7 or day 10 according to the manufacturer’s protocol. CDK6 activity assay in vitro A measure of 100 ng of GST-p18 protein (GST-p18 protein was expressed and purified in our lab) was diluted in kinase buffer (5 mM MOPS, pH 7.2, 2.5 mM glycerol 2-phosphate, 5 mM MgCl 2 , 1 mM EGTA, 0.4 mM EDTA, 0.05 mM DTT and 50 ng μl −1 BSA), and pre-incubated with/without the P18INs compounds (0.5 μM) at room temperature for 30 min, and then mixed with 200 ng of CDK6/CyclinD1 complex (Sigma, C1374) and 2 μg of GST-Rb (Sigma, SRP0256). Each reaction was initiated with the addition of 2.0 μCi of [γ-32P]ATP, bringing the final volume to 30 μl. The mixture was incubated at 30 °C for 60 min and the reaction was terminated by spotting the mixture onto polyvinylidene difluoride membrane paper. After washing, 32P-labelled GST-Rb was quantitatively analysed by a scintillation counter (LS6500; Beckman Coulter). Virtual screening for chemical inhibitors of the p18 protein 3D structures of the p18 protein were modelled based on X-ray crystal structures of free p18 (PDB entry: 1IHB) and the p18/CDK6 complex (PDB entry: 1G3N) [20] , [37] by using our reported protein modelling protocol [18] . The putative p18-binding cavities were defined by using a solvent-accessible surface calculation algorithm [17] based on the interface contacting residues known from X-ray crystallography and site-directed mutations. 3D chemical database virtual screenings were conducted using our reported docking virtual screening/CScore algorithm [17] to identify small molecules that can interfere with the p18/CDK6-binding cavity. All computations were performed on a dual-core dual-CPU Xeon-based HPCC 30-processor Dell cluster, loaded with TriposSybyl molecular modelling package (version 1.3). Chemistry and compounds P18IN011 was synthesized in house while others were purchased from the Maybridge Company. The chemical compound of P18IN003 is 4,5-bis(4-methoxyphenyl)-1,5-dihydroimidazol-2-one, which is a R/S racemic. 1 H NMR (400 MHz, DMSO- d 6 ): δ 10.27 (s, 1H), 7.25–7.23 (m, 4H), 6.90–6.88 (m, 4H), 3,75 (s, 6H); 13 C NMR (400 MHz, DMSO- d 6 ): δ =158.8, 154.5, 128.7, 123.3, 117.2, 114.5, 55.6; HRMS ( m / z ): [M+H] + calculated (calcd) for C 17 H 17 N 2 O 3 , 297.1234; found, 297.1237. P18IN011 is 1,2-benzoxazol-3-yl 4-acetamidobenzenesulfonate ( Supplementary Fig. 5 ). 1 H NMR (400 MHz, DMSO- d 6 ): δ =10.57 (s, 1H), 8.00–7.97 (m, 2H), 7.90–7.87 (m, 2H), 7.83–7.74 (m, 2H), 7.69–7.66 (m, 1H), 7.50–7.46 (m, 1H), 2.12 (s, 3H); 13 C NMR (400 MHz, DMSO- d 6 ): δ =170.0, 164.7, 160.3, 146.4, 132.5, 130.9, 126.4, 125.7, 121.3, 119.4, 113.9, 111.5, 24.7; HRMS ( m / z ): [M+H] + calcd for C 15 H 13 N 2 O 5 S, 333.0540; found, 333.0552. P18IN003a is 1-[2-[3-[[2-(benzoyl)-4-chlorophenyl]amino]-2-hydroxypropoxy]-5-chlorophenyl]ethanone. 1 H NMR (400 MHz, DMSO- d 6 ): δ =8,63 (t, J =5.2, 1H), 7.64–7.53 (m, 7H), 7.48–7.45 (m, 1H), 7.28–7.22 (m, 2H), 6.99 (d, J =9.2, 1H), 5.57 (d, J =4.4, 1H), 4.18–4.12 (m, 3H), 3.57–3.52 (m, 1H), 3,38–3,36 (m, 1H), 2.61 (s, 3H); 13 C NMR (400 MHz, DMSO- d 6 ): δ =198.2, 197.6, 157.0, 150.4, 139.7, 135.1, 133.6, 133.5, 131.8, 129.7, 129.2, 129.0, 128.9, 125.0, 118.2, 117.5, 116.0, 114.7, 71.9, 67.5, 45.9, 32.2; HRMS ( m / z ): [M+H] + calcd for C 24 H 22 Cl 2 NO 4 , 458.0920; found, 458.0931. P18IN004 is N -acetyl-4, 4′-diaminodiphenylsulfone. 1 H NMR (400 MHz, DMSO- d 6 ): δ =10.30 (s, 1H), 7.77–7.71 (m, 4H), 7.52–7.50 (m, 2H), 6.62–6.60 (m, 2H), 6.12 (s, 2H), 2.07(s, 3H); 13 C NMR (400 MHz, DMSO- d 6 ): δ =169.5, 153.9, 143.4, 137.3, 129.6, 128.2, 126.6, 119.3, 113.4, 24.6; HRMS ( m / z ): [M+H] + calcd for C 14 H 15 N 2 O 3 S, 291.0798; found, 291.0805. P18IN005 is 2-butylamino-1-(4-methoxyphenyl)-2-phenylethanone. 1 H NMR (400 MHz, DMSO- d 6 ): δ =9.46 (s, 1H), 8.04–8.02 (m, 2H), 7.59–7.58 (m, 2H), 7.48–7.42 (m, 3H), 7.05 (d, J =9.2, 2H), 6.35 (s, 1H), 3,83 (s, 3H), 2.85–2.68 (m, 2H), 1.70–1.62 (m, 2H), 1.33–1.27 (m, 2H), 0.87 (t, J =7.6, 3H); 13 C NMR (400 MHz, DMSO- d 6 ): δ =191.7, 164.7, 132.6, 132.1, 130.5, 130.0, 129.7, 126.3, 114.9, 64.6, 56.2, 45.7, 27.8, 19.8, 13.9,; HRMS ( m / z ): [M+H] + calcd for C 19 H 24 NO 2 , 298.1802; found, 298.1803. All compounds were prepared in DMSO stock solution at a concentration of 20 mM and stored at −20 °C before use. The compounds were then diluted in Iscove’s modified Dulbecco’s medium (GBICO) to make a working solution, as needed. The final DMSO concentration was less than 0.1% in the working solution. Statistical analysis Tests of statistical significance were performed using a two-tailed Student’s t -test. Standard deviation was used to determine the error bars shown in the figures. How to cite this article: Gao, Y. et al . Small-molecule inhibitors targeting INK4 protein p18 INK4C enhance ex vivo expansion of haematopoietic stem cells. Nat. Commun. 6:6328 doi: 10.1038/ncomms7328 (2015).